Heterovalent cation substitutional doping for quantum dot homojunction solar cells Colloidal quantum dots have emerged as a material platform for low-cost high-performance optoelectronics. At the heart of optoelectronic devices lies the formation of a junction, which requires the intimate contact of n-type and p-type semiconductors. Doping in bulk semiconductors has been largely deployed for many decades, yet electronically active doping in quantum dots has remained a challenge and the demonstration of robust functional optoelectronic devices had thus far been elusive. Here we report an optoelectronic device, a quantum dot homojunction solar cell, based on heterovalent cation substitution. We used PbS quantum dots as a reference material, which is a p-type semiconductor, and we employed Bi-doping to transform it into an n-type semiconductor. We then combined the two layers into a homojunction device operating as a solar cell robustly under ambient air conditions with power conversion efficiency of 2.7%. Doping of bulk semiconductors has enabled a vast majority of functionalities that we experience today from transistors, to light-emitting diodes and photovoltaics. A new class of solution-processed semiconductors, which are of colloidal quantum dots (QDs), has been introduced some 30 years ago, and since then dramatic progress in the control of optical and electronic properties has enabled functionalities that are offered previously by bulk semiconductor with the added benefits of solution processability and facile bandgap tunability. Exquisite control over the shape, stoichiometry and composition of QDs has allowed for the demonstration of highly performing solar cells, light-emitting diodes and photodetectors [1] , [2] , [3] , [4] . Doping of QDs lies at the heart of achieving new functionalities that are currently being offered by single crystalline semiconductors [5] , [6] . The development of junctions based on QDs is instrumental to achieve high-performance solar cells and photodetectors, as it has been in the case of single crystalline semiconductors. Preliminary attempts to dope QDs were based on remote doping schemes in which ligand molecules served the purpose of the dopant [7] , [8] . Ligands have also been utilized to passivate the surface of the dots allowing for n-type doping in PbSe QDs from the excess of Pb cations, leading to p- and n-type field effect transistors [9] . More recently, the incorporation of substitutional and interstitial doping using heterovalent atoms has been proposed as a method for heavily doped semiconductor InAs QDs and their effect on the optical properties, and the density of states has been thoroughly studied [10] . For chalcogenide dots of divalent cations, such as PbS and CdSe, p-type doping has been achieved with the addition of Ag 1+ , which is believed to replace Pb 2+ and Cd 2+ , respectively, thus providing positive free carriers [11] , [12] . However, since PbS dots are typically p-type, because of oxidation of their surface, a more intriguing task would be to dope them n-type especially considering the technological applications of this material [13] . Recently and in contrast to the aforementioned cation-doping approaches, stoichiometry control was employed as a means to tune doping in QD solids [14] . N-type doping of PbS was achieved by substitution of S 2− with monovalent halide ions resulting in free electrons [15] , [16] , [17] from the excess of Pb atoms in PbS QDs. This methodology has been utilized successfully for the creation of PbS QD homojunctions for high-efficiency photovoltaics [16] . In another report, the evaporation of excess cations or anions on QD films has shown to tailor the doping profile accordingly. Excess of anions leads to higher p-type doping profiles, whereas excess of cations leads to n-type doping as monitored by field effect transistor measurements [18] , but without any demonstration in optoelectronic devices. Relying on Pb atoms for the n-type doping has been reported to suffer from oxidation effects since the excess Pb atoms upon exposure to ambient air transform from electron-donating moiety near the conduction band to electron acceptor near the valence band turning the material into p-type. During the revision of the current manuscript, another doping scheme based on charge transfer from cobaltocene to PbS(e) QDs was reported [19] . This was based on charge transfer from cobaltocene molecules to the conduction band states of QDs that allowed the demonstration of absorption bleaching in the heavily doping regime. However, robust functional optoelectronic devices based on this approach have yet to be demonstrated. In sum, a robust doping scheme for functional homojunctions that can operate under ambient environmental conditions still remains a challenge. We took the view that to develop a robust doping scheme we would have to employ a heterovalent substitutional doping methodology in which the excess electrons would be provided by the excess electrons offered by the valency of the dopant atoms. We posited that this dopant atom would have to possess at least an excess electron available for donation and an atomic radius similar to the original cation of Pb. Bismuth is an element with +3 valency and atomic radius similar to that of Pb; to test our hypothesis, we added bismuth acetate in the standard lead-oleate precursor method used for producing oleic acid-capped PbS dots [20] . In this method, PbS dots are synthesized in an acidic environment and incorporation of bismuth in the dots is expected to be favoured in accordance with the hard–soft acid–base theory as this has been extensively discussed in other works concerning QD cation-exchange reactions [21] . Our results confirm that bismuth is efficiently incorporated in the PbS QDs and suggest that it acts as an electron donor, influencing the QDs’ optoelectronic properties and rendering them suitably n-type as to be utilized in air-stable homojunction and Schottky junction solar cells. Optical properties and material characterization of QDs We synthesized a range of Bi-doped PbS dots, with nominal atomic Bi/Pb precursor ratios from 0.1 to 4.5%. Inductively coupled plasma optical emission spectrometry (ICP-OES) analysis of our samples shows highly efficient incorporation of Bi in the dots with accompanied replacement of Pb as indicated by the evolution of the measured Bi/Pb ratio shown in Fig. 1a (for clarity of discussion and unless otherwise specified from now on we will refer to precursor Bi/Pb % ratios to describe our doped materials). Transmission electron microscopy (TEM) investigation of neat and Bi-doped QDs (Bi/Pb=3.2%) suggests that their morphology (shape and size) has not been altered markedly showing average diameters of ~3.5±0.3 nm ( Fig. 1b and Supplementary Figs S1–S5 )). 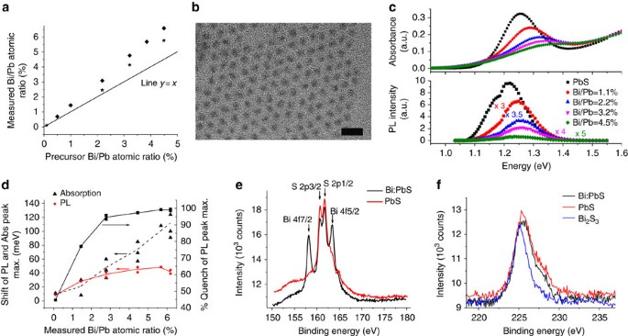Figure 1: Optical properties and material characterization of Bi-doped PbS QDs. (a) Measured from ICP-OES Bi/Pb atomic ratio of QDs as a function of nominal precursor ratio. Different symbols indicate different sets of samples. Line represents a hypothetical 1:1 relationship between measured and precursor ratios. (b) TEM image of Bi:PbS (Bi/Pb=3.2%) QDs (10 nm scale bar). (c) Typical optical absorption and photoluminescence spectra of reference PbS and Bi:PbS QDs at 5 g l−1in toluene (all have a size of 3.5±0.3 nm as measured from TEM images). (d) Measured shifts of excitonic absorption and photoluminescence peaks and quenching of the later of Bi:PbS with respect to reference PbS QDs, as a function measured from ICP-OES Bi/Pb ratios (average ratios where applicable). Lines in the graph are guides to the eye. (e) XPS spectral regions of Bi4f and S2p for PbS and Bi:PbS QDs (precursor Bi/Pb=3.2%) and (f) the XPS spectral region of S2s of the same samples as inFig. 1eas well as Bi2S3nanocrystals28, demonstrating the absence of a distinct bismuth sulphide feature for the case of Bi:PbS QDs. Figure 1: Optical properties and material characterization of Bi-doped PbS QDs. ( a ) Measured from ICP-OES Bi/Pb atomic ratio of QDs as a function of nominal precursor ratio. Different symbols indicate different sets of samples. Line represents a hypothetical 1:1 relationship between measured and precursor ratios. ( b ) TEM image of Bi:PbS (Bi/Pb=3.2%) QDs (10 nm scale bar). ( c ) Typical optical absorption and photoluminescence spectra of reference PbS and Bi:PbS QDs at 5 g l −1 in toluene (all have a size of 3.5±0.3 nm as measured from TEM images). ( d ) Measured shifts of excitonic absorption and photoluminescence peaks and quenching of the later of Bi:PbS with respect to reference PbS QDs, as a function measured from ICP-OES Bi/Pb ratios (average ratios where applicable). Lines in the graph are guides to the eye. ( e ) XPS spectral regions of Bi4f and S2p for PbS and Bi:PbS QDs (precursor Bi/Pb=3.2%) and ( f ) the XPS spectral region of S2s of the same samples as in Fig. 1e as well as Bi 2 S 3 nanocrystals [28] , demonstrating the absence of a distinct bismuth sulphide feature for the case of Bi:PbS QDs. Full size image Despite no significant change in morphology, doping has a profound impact on the excitonic optical properties of the material as seen in Fig. 1c,d . The position of the first excitonic phototransition monotonically shifts to higher energies. The blue shift Δ E of the excitonic absorption scales as Δ E ~ N 1.1±0.2 , where N is measured Bi/Pb in % (which translates to elemental doping density), much stronger compared with Δ E ~ N 2/3 , which is predicted by the standard Burstein–Moss effect for bulk semiconductors [22] . This difference can in part be associated with the confinement of charge impurities in small QDs, its impact on the density of the states’ distribution and the formation of Urbach tailing in the confined states [10] . In addition to the observed blue shift, we also noticed a progressive quenching of the excitonic feature with increasing Bi-doping. This can be because of effective filling with electrons of 1S e as reported also in the case of cobaltocene doping [19] , the distortion of the crystal structure because of incorporation of bismuth and thus the lowering of the oscillator strength, or the combination of both mechanisms. The excitonic optical emission is blue shifted, although not as strongly as the absorption shift. Most profoundly, however, the emission strength is quenched by more than 94% for Bi/Pb ratios higher than 2%. This has been observed in charged and doped QDs and is attributed to strong local electric fields and Auger recombination, respectively [23] , [24] . These effects, taken together, are signatures of doping that have been reported to arise from the perturbation of the density of states after dopant incorporation [10] and filling of optically accessible states of QDs [19] . To gain additional insights on the incorporation of bismuth in the PbS QDs, we performed X-ray photoelectron spectroscopy (XPS) on films prepared via a layer-by-layer spin-casting method in ambient atmosphere including ligand exchange with 1,2-ethanedithiol (EDT) as used for the devices presented subsequently. As opposed to reference PbS QDs films, the spectrum ( Fig. 1e ) of a doped sample (Bi/Pb=3.2%) contains the bismuth 4f doublet peak in a spectral region that also includes three S2p doublets associated with PbS, bound and unbound thiols [25] . (Detailed analysis of XPS spectra is presented in Supplementary Figs S6,S7 and Supplementary Tables S1 and S2 ). Deconvolution of the overall region indicates that Bi doublets (158.3 and 163.5 eV) are associated with Bi-S bonds as closely referenced (0.1 eV difference) to bismuth sulphide (Bi 2 S 3 ) [26] and that there is no secondary bismuth phase such as metallic Bi or its oxides. Analysis of sulphur 2s spectrum ( Fig. 1f ) shows that it can be deconvoluted to two peaks at 225.4 and 227.5 eV attributed, respectively, to PbS and thiolate [27] . A distinct signature of Bi 2 S 3 in the sulphur peak can be elusive because of its overlap with the peaks associated to PbS and thiolates, given the particularly low doping ratio. Quantitative analysis of the XPS data indicates that bismuth incorporation is accompanied by an almost equivalent drop of the Pb content, retaining the total cation/S atomic ratio at 0.95 for both pure and doped dots. This analysis is in close agreement to the ICP-OES result regarding the Bi/Pb ratio for the same sample, 4.1% and 5.4% respectively for the two techniques. X-ray diffraction (XRD) characterization of these materials (see Supplementary Fig. S8 , Supplementary Table S3 and Supplementary Note 1 ) has shown that the introduction of Bi does not induce an alteration of the crystal structure of PbS. However, it leads to a crystal distortion manifested by an increase in the lattice constant (by 0.02–0.03 Å for Bi/Pb=4.5%) with increasing doping density as observed by the position of the reflections of the crystal planes. Although the exact position of Bi atoms within the PbS QD cannot be determined (because of the similar atomic mass of the two elements), this study suggests the incorporation of bismuth in the PbS QD structure by substitution of lead. Electronic properties of doped QD films and homojunctions We now turn to the optoelectronic properties of the doped QDs and their employment in QD homojunctions intended for solar cell applications. Their n-type character is demonstrated by the formation of photovoltaic p-n diodes formed between doped and pure QDs. Two architectures, the normal and the inverted homojunction schematically shown in Fig. 2a , were investigated. The choice of the different top ohmic contact electrode for each case was based on control Schottky-type devices, which demonstrate that the p- and n-type QDs form different types of contacts for the same electrode material (see Supplementary Figs S9–S14 and Supplementary Notes 2 and 3 for further description of Schottky studies). 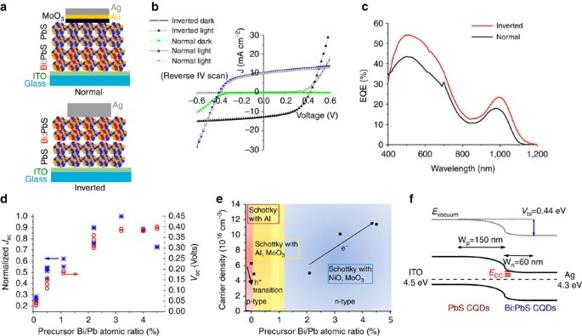Figure 2: Electronic properties of Bi-doped PbS QDs and homojunctions with PbS QDs. (a) Schematic illustration of the normal and inverted QD-homojunction solar cell geometries. (b) Typical J-V curves of normal (ITO/Bi: PbS (50 nm)/PbS (200 nm)/MoO3/Au/Ag) and inverted (ITO/PbS (150 nm)/Bi:PbS (75 nm)/Ag) homojunctions at dark and at 100 mW cm−2AM1.5 solar light and (c) EQE spectra of the cells showing efficient photoresponce in Vis-IR. (d) Comparison ofJscandVocof normal homojunctions as a function of precursor Bi/Pb ratios for doped QDs. Multiple points refer to multiple device pixels. (e) Summary of ability to form a Schottky junction with different electrode materials and carrier density and type as estimated by Mott–Schottky analysis of Schottky-type devices, as a function of doping concentration. (f) Schematic band diagram of inverted cell with estimatedVbiand depletion widths within p- and n-type layers. Figure 2: Electronic properties of Bi-doped PbS QDs and homojunctions with PbS QDs. ( a ) Schematic illustration of the normal and inverted QD-homojunction solar cell geometries. ( b ) Typical J-V curves of normal (ITO/Bi: PbS (50 nm)/PbS (200 nm)/MoO3/Au/Ag) and inverted (ITO/PbS (150 nm)/Bi:PbS (75 nm)/Ag) homojunctions at dark and at 100 mW cm −2 AM1.5 solar light and ( c ) EQE spectra of the cells showing efficient photoresponce in Vis-IR. ( d ) Comparison of J sc and V oc of normal homojunctions as a function of precursor Bi/Pb ratios for doped QDs. Multiple points refer to multiple device pixels. ( e ) Summary of ability to form a Schottky junction with different electrode materials and carrier density and type as estimated by Mott–Schottky analysis of Schottky-type devices, as a function of doping concentration. ( f ) Schematic band diagram of inverted cell with estimated V bi and depletion widths within p- and n-type layers. Full size image The two types of homojunctions have opposite polarities at dark and under AM1.5 illumination while presenting similar short-circuit currents ( J sc ) and open circuit voltages ( V oc ) values as seen in Fig. 2b . The figures of merit under AM1.5 illumination for the inverted homojunction shown are as follows: V oc =0.42 V, J sc =12.8 mA cm −2 , fill factor=50% and power conversion efficiency of 2.7% (see Supplementary Fig. S15 for further data on devices). Photon-to-electron conversion in these devices occurs over the full spectrum of the QD optical absorption ( Fig. 2c ). This broadband photoresponse originates from both the p- and the n-type layers as also indicated by the EQE spectra ( Supplementary Figs S9,S11 ) of respective Schottky-type devices, proving the optoelectronically active nature of the doped PbS QDs. The effect of doping on the optoelectronic properties of the homojunctions was further studied by comparing the J sc and V oc values of homojunctions made of n-type Bi:PbS of different Bi/Pb ratios as shown in Fig. 2d . With Bi/Pb ratio increasing to 2%, the n-type character of doped dots and thus V oc and J sc of the homojunctions are markedly improved, whereas heavier doping to 4.5% Bi/Pb leads to less pronounced increase in V oc and a reduction in J sc . Doping of 0.1% leads to a reduction in hole carrier density pointing to a still p-type but less doped film. The transition from a p-type to an n-type character of the QDs occurs for doping concentrations of ~0.5–1% as observed by the ability of these films to form Schottky junctions with both aluminium and MoO 3 , as indicated in Fig. 2e (see also Supplementary Fig. S12 ). It should be noted here that Schottky devices with 0.5–1% Bi-doping did not yield appreciable changes in the capacitance with reverse bias, even in very thick films; thus, the carrier density could not be determined by the slope of the Mott–Schottky plot. We call this a transition region in which we believe that Bi atoms compensate the p-type dopants of the PbS QDs and progressively lead to transforming them into n-type at higher Bi-doping concentration. The direct correlation between increasing dopant density and electron concentration of the n-type QDs is further explored from Mott–Schottky analysis (method described in Supplementary Note 3 ) of the capacitance–voltage characteristics of NiO/Bi:PbS junctions as shown in Fig. 2e and Supplementary Fig. S9 . The same analysis of Bi:PbS/MoO 3 ( Supplementary Fig. S13 ) and Bi:PbS/PbS ( Supplementary Fig. S16 ) junctions for Bi/Pb>3% inferred similar electron concentration values: 1 × 10 17 and 1.4 × 10 17 cm −3 , respectively. The n-type QDs are thus more heavily doped than the p-type PbS, which yield ~6.2 × 10 16 cm −3 carrier density ( Supplementary Fig. S14 ). This reflects upon the distribution of the depletion region across the p-n interface of the homojunctions, as also studied by monitoring the electronic characteristics of diodes with varying p- and n-layer thicknesses ( Supplementary Tables S4,S5 and Supplementary Figs S16,S17 ). Figure 2f schematically illustrates that most of the depletion region lies within the p-type layer. The built-in potential V bi , measured by the intersection between the light and dark IV curves of the junctions at forward bias, as well as analysis of their CV characteristics [29] , at room temperature, is estimated to be ~0.44 eV. The formation of a built-in potential ( V bi ) at the homojunctions’ interface arises from the relative shift of the Fermi levels ( E F ) of the p- and n-type layers with respect to vacuum (zero) energy. In order to explore the effect on the Fermi level that Bi-doping has in our PbS QDs, and to support our hypothesis for n-type doping, we performed UV photoelectron spectroscopy (UPS) measurements. 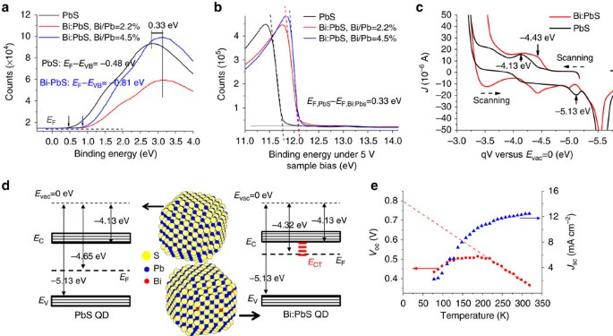Figure 3: Impact of doping on electronic structure of QDs. (a) UPS (UV excitation by HeI=21.21 eV) valence band-onset spectral region and measuredEF−EVBdifferences for PbS and two Bi:PbS unbiased QD thin film samples, and (b) cutoff region of the spectra with the samples biased at −5 V, including measuredEFshift by doping. (c) Part of cyclic voltammetry graphs at dark for PbS and Bi:PbS (precursor Bi/Pb=3.2%) QDs. Marked by arrows are the positions of the first oxidation and reduction peaks attributed to the valence band (HOMO) at −5.13 eV and conduction band (LUMO) at −4.13 eV of PbS, respectively. Thexaxis is the energy product of the elementary charge and applied voltage, referenced againstEvac=0 using the ferrocene/ferrocenium couple. For Bi:PbS (Bi/Pb=3.2%) an additional conduction tailEcT(0.3 eV below LUMO) reduction peak at 4.43 eV and a mirror oxidation one during the reverse scan, are observed. (d) Comparison of theEV,EClevels as measured by cyclic voltammetry for pure and doped QD films with 1 eV bandgap (with broadening due to size distribution of single dots).EVis constant with respect to vacuum and the Fermi levels are positioned with respect toEVaccording to UPS. The crystal models of PbS and Bi:PbS QDs of 3.6 nm diameter, consisting of x6 rock-salt unit cells in each direction and truncated at their {110} and {111} edge and corner planes, respectively, indicate that a doped QD with Bi/Pb=4.5% contains ~728 and 33 atoms of Pb and Bi, respectively, assuming that Bi substitutes Pb. (e) Dependence ofVocandJscof an inverted homojunction on temperature with extrapolation of linearVoc-T regions towards T→0 K. Figure 3a shows the difference in the Fermi level from the valence band level of the two materials. The Fermi level of PbS QDs is 0.48 eV from the valence band, whereas the Bi-doped PbS has an energy offset of 0.81 eV. This yields a Fermi level difference between the two materials of 0.33 eV as supported by the cutoff spectra measurement shown in Fig. 3b . Although this value is in accordance with other reports of UPS measurements on PbS QDs [30] , it is lower than the experimentally measured value in working homojunction solar cells. The origin of this difference is because of the fact that UPS measurements take place at very high vacuum conditions. Neat PbS QDs are known to become p-type-doped because of phys- and chem-adsorbed species of moisture and oxygen in working devices. Thus, in the presence of oxygen the PbS Fermi level is found to be ~4.8–4.9 eV (ref. 31 ), as supported by Kelvin Probe measurements. This in turn would result in a Fermi level difference of ~0.48 eV with respect to Bi-doped PbS in agreement with the experimental values from electronic characterization. Figure 3: Impact of doping on electronic structure of QDs. ( a ) UPS (UV excitation by HeI=21.21 eV) valence band-onset spectral region and measured E F − E VB differences for PbS and two Bi:PbS unbiased QD thin film samples, and ( b ) cutoff region of the spectra with the samples biased at −5 V, including measured E F shift by doping. ( c ) Part of cyclic voltammetry graphs at dark for PbS and Bi:PbS (precursor Bi/Pb=3.2%) QDs. Marked by arrows are the positions of the first oxidation and reduction peaks attributed to the valence band (HOMO) at −5.13 eV and conduction band (LUMO) at −4.13 eV of PbS, respectively. The x axis is the energy product of the elementary charge and applied voltage, referenced against E vac =0 using the ferrocene/ferrocenium couple. For Bi:PbS (Bi/Pb=3.2%) an additional conduction tail E c T (0.3 eV below LUMO) reduction peak at 4.43 eV and a mirror oxidation one during the reverse scan, are observed. ( d ) Comparison of the E V , E C levels as measured by cyclic voltammetry for pure and doped QD films with 1 eV bandgap (with broadening due to size distribution of single dots). E V is constant with respect to vacuum and the Fermi levels are positioned with respect to E V according to UPS. The crystal models of PbS and Bi:PbS QDs of 3.6 nm diameter, consisting of x6 rock-salt unit cells in each direction and truncated at their {110} and {111} edge and corner planes, respectively, indicate that a doped QD with Bi/Pb=4.5% contains ~728 and 33 atoms of Pb and Bi, respectively, assuming that Bi substitutes Pb. ( e ) Dependence of V oc and J sc of an inverted homojunction on temperature with extrapolation of linear V oc -T regions towards T→0 K. Full size image Despite the heavily doped PbS QDs, utilizing a Bi/Pb ratio of ~3–5%, which would in theory yield doping densities on the order of 10 20 cm −3 , in our optoelectronic measurements we observe much lower effective carrier densities on the order of 10 17 cm −3 and the corresponding Fermi level position that is not in accordance with degenerate doping. A similar effect has also been observed in anionic doping in PbS QDs [16] , [17] and has been attributed to the formation of band-tail states below the conduction band ( E CT ) resulting from pre-existing surface-dangling bonds and lattice dislocations or distortion by the introduction of the dopant atoms. A significant proportion of the donating electrons of the dopants has then to be allocated for filling these electron states. We employed cyclic voltammetry (C-V) to monitor this effect in our structures, and in Fig. 3c we plot the C-V plots for the cases of PbS and Bi:PbS QD films. The C-V plot reveals a redox pair of peaks appearing within the bandgap near the conduction band at ~4.4 eV. The nature of this peak indicates the presence of available electronic states that can now be partially filled by the donation of electrons from Bi atoms, and which determine the position of the Fermi level. Figure 3d summarizes the findings from C-V and UPS regarding the energy positions of E V , E C and E F of pure and doped materials and considering that the electronic bandgap of the QD films is ~1 eV as determined from the cutoff regions of EQE spectra of Schottky and p-n devices at 1,200 nm ( Supplementary Figs S9,S11 ). This refers to dots with Bi/Pb=4.5% and the shown crystallographic representations of the dots give an approximate estimate on the actual number of dopant atoms for such a quasi-spherical 3.6-nm dot corresponding to ~33 Bi atoms. The presence of the E CT states is expected to affect the maximum achievable V oc of a homojunction. In order to explore this effect, we monitor the V oc dependence of the junction as a function of temperature as shown in Fig. 3e . At progressively decreasing temperature, the donated electrons that populate the E CT states freeze-out pinning the Fermi level of the n-type material within the E CT distribution. Extrapolation of the linear part of the V oc versus T dependence to 0 K, points to a maximum achievable V oc from this system of ~0.8 V, determined by the Fermi level splitting of the p-type and n-type materials in the presence of interface recombination [32] . Heterovalent cation substitutional doping has been presented as a promising means to develop functional optoelectronic devices, demonstrated by the development of a QD-homojunction solar cell. Our devices are fabricated and tested in ambient air showing significant robustness—a prerequisite for the commercialization of nanocrystalline solar cells and a flagship benefit over organic material platforms. The current approach of atomic doping is readily applicable either in situ during the growth of the nanocrystals or post synthetically (see Supplementary Figs S18,S19 and Supplementary Note 4 ). This methodology taken together with recent advances in atomic passivation schemes [33] can lead to significant improvement of maximum attainable V oc via passivation of the deepest E CT states allowing for higher effective doping densities to be reached. Chemicals Lead (II) oxide (99.999%), hexamethyldisilathiane (TMS) (synthesis grade), 1-octadecene (technical grade 90%), oleylamine (technical grade 90%), EDT (technical grade >90%) and toluene (anhydrous, 99.8%) were purchased from Sigma Aldrich. Bismuth (III) acetate (99.999%, metals basis) was purchased from Alfa Aesar. Acetone, acetonitrile and methanol were purchased from Panreac. Synthesis of PbS and Bi-doped PbS QDs Oleic acid-capped PbS QDs with a first excitonic peak at 900–980 nm were synthesized with a modified version of a standard method [20] , using a standard Schlenk line as follows: 0.45 g of PbO was dissolved in 1.5 ml oleic acid and 3 ml octadecene under vacuum (0.2 × 10 −1 mbar) overnight (16 h) at 95 °C. Afterwards, 15 ml of octadecene were further added. Then, under Ar atmosphere, temperature was raised to 120 °C, and 0.21 ml TMS in 10 ml octadecene were injected, and the final solution was left to cool down to 36 °C. Then QDs were isolated/purified by precipitation upon the addition of excess acetone, centrifugation and re-dispersion in toluene in normal atmospheric conditions. This cleaning process was repeated twice. Bi:PbS QD synthesis was performed in the same way, with the addition of the appropriate amount of bismuth acetate in the original lead-precursor solution. For a typical synthesis of Bi:PbS with precursor Bi/Pb=3.2%, we added 0.025 g bismuth acetate. Thin film and device fabrication Prior to thin-film fabrication, QD/toluene stock solutions were transferred to a nitrogen glovebox, where oleylamine was added to them (1.5 ml oleylamine for ~120 g per l.3 ml stock solution). After 2 days, the solutions were taken out of the glovebox and the QDs were further purified by two rounds of precipitation with methanol/centrifugation/re-dispersion in toluene. QD inks of 30 g l −1 QD/toluene were used for thin-film fabrication. Semiconducting QD thin films were fabricated on 12.5 × 12.5 mm glass/ITO substrates by spin-coating using a layer-by-layer approach employing ligand exchange on the dots’ surface with EDT inside a fume hood. Each layer is deposited as follows: two drops of QD ink were dropped on a static substrate on the spin coater. Then the substrate was set to spin at 2,000 r.p.m. After 20 s, the substrate was rinsed with three drops of 2% EDT in acetonitrile solution, and 30 s later with 6–10 drops of acetonitrile, and 10 s later with 6–10 drops of toluene. The spinning was stopped and the process was repeated for achieving the desired layer thickness. Each spin-casting cycle yields approximately a 25-nm thick layer. Different QD materials were deposited on top of each other using the same process. For the device fabrication, the films were left to dry overnight in a nitrogen glovebox, and then transferred out of it for top contact deposition using a Kurt J. Lesker NANO36 evaporator. Typical evaporation parameters for different materials were as follows: 8 nm MoO 3 (Sigma Aldrich) deposited at 0.1 Å s −1 , 40 nm Au at 1 Å s −1 , 140 nm Ag at 1.5 Å s −1 , 0.8 nm LiF at 0.1 Å s −1 and 160 nm Al at 1–2 Å s −1 . NiO (5 nm) was deposited on ITO by RF sputtering. Top electrodes were either of 2 mm-diameter circular geometry when plain ITO substrate was used, thus defining a 3.14-mm 2 pixel device, or 2-mm-width striped geometry when substrates of perpendicular to top contact 2-mm-wide ITO stripes were used, thus defining 4-mm 2 rectangular devices. Devices of those different geometries/sizes perform the same. After fabrication, devices were commonly stored in open air for at least 1 day before being tested. Material characterization Absorption spectra of 5 g l −1 QD/toluene solutions were measured with a Varian 5000 UV–vis-NIR spectrophotometer. The photoluminescence (PL) spectra were obtained using a Renishaw inVia Raman microscope. Very thick drop-cast samples (from ~120 g l −1 QD/toluene solutions) of PbS and Bi:PbS nanocrystals of varying Bi concentrations were irradiated with a 785-nm laser using the same neutral density filter; the measured Raman spectrum from 100 to 5,000 cm −1 with a resolution of 0.6 cm −1 , as a shift from the 785-nm laser line, was converted to wavelength in nanometres. Raman spectroscopy for crystal phase identification was performed with the aforementioned Raman microscope using 532-nm laser excitation. Results regarding PL quenching were further confirmed by PL measurements of QD/toluene solutions of same concentration (0.4 g l −1 ) acquired with a Horiba JobinYvon iHR550 fluorolog system equiped with a Hamamatsu R5509-73 photomultiplier tube detector. Transmission electron microscopy for samples made by drop-casting very thin QD solutions on lacey carbon films was performed with a JEOL 2100 microscope operated at 200 kV and with a FEI Tecnai F30 microscope equipped with a field emission gun and operated at 300 kV. Scanning TEM images in high-angle annular dark-field mode were acquired in an FEI Titan 60–300 microscope operated at 300 kV and equipped with a probe aberration corrector to provide a spatial resolution below 1 Å. XRD spectroscopy on several micron-thick QD films, which were additionally flattened by pressing against a glass surface, was performed using a Panalytical XPERT-PRO diffractometer equipped with Cu K-alpha (1.540598 Å) source and operated at a continuous mode with a 0.0394deg step size. C-V measurements were performed in 0.1 M tetrabutylammonium perchlorate in acetonitrile solution using a CH instruments electrochemical workstation system employing a standard three-electrode electrochemical cell under nitrogen purge. Five microlitre of a 10 g l −1 toluene solution were placed on a platinum working electrode and dried. Next, the working electrode was dipped in a 2% vol. EDT solution in acetonitrile for 20 s. The scan range was set to −2 to 2 V and scan speed was set to 0.1 V s −1 starting towards reduction potentials. Silver/silver nitrate (0.1 M) in acetonitrile reference and platinum wire counter electrodes were calibrated against ferrocene as an internal reference of the system (0.64 V versus standard hydrogen electrode). Energy levels with respect to vacuum energy were calculated from the potential of the standard hydrogen electrode (4.44 eV), similar to other studies [34] . XPS experiments under ultrahigh vacuum (10 −8 –10 −9 Torr) were performed in a PHI 5500 Multitechnique System (from Physical Electronics) with a monochromatic X-ray source (Aluminium Kalfa line of 1,486.6 eV energy and 350 W), placed perpendicular to the analyser axis and calibrated using the 3d5/2 line of Ag with a full-width at half maximum of 0.8 eV. The analysed area was a circle of 0.8 mm diameter, and the selected resolution for the spectra of the different elements was 23.5 eV of pass energy and 0.1 eV per step. For chemical analysis, the binding energy was further calibrated using 284.8 eV as the value of C1S peak position. Samples for XPS and UPS were 150-nm thick QD films on ITO prepared in the same way as thin films for devices. XPS spectra were analysed using Shirley backgrounds (except for the Bi4f and S2p for which a linear background was used), and the energy scales were calibrated using the C1s peak at 284.8 eV. The amount of Pb was measured using the Pb4f spectral region. Each Pb4f spectrum was deconvoluted to two peaks at 137.6 and 142.5 eV, with a 4:3 area ratio between them, corresponding to the Pb4f doublet of PbS. The amount of sulphur, oxygen and carbon was measured using the S2s, O1s and C1s spectral regions. The amount of Bi was measured using the Bi4f spectral region. The Bi4f spectral region overlaps with the S2p region. The Bi4f signal is deconvoluted to a single doublet (158.3 and 163.5 eV) with a peak ratio of 4:3. The energy of this doublet is close (difference is 0.1 eV) to reported values for Bi 2 S 3 (ref. 26 ). In order to prevent erroneous estimation of Bi, the S2p signal was also analysed using three doublets at 160.7, 161.8 and 163.5 eV corresponding to PbS, bound thiols and unbound thiols, respectively, similar to previous works [25] , [35] . The two peaks of each doublet are distant by 1.2 eV and have peak ratio of 2:1. All the deconvoluted spectra for PbS and Bi:PbS (precursor Bi/Pb=3.2%) QDs used for XPS chemical analysis are shown in Supplementary Figs S6,S7 with peak details within them. UPS measurements were performed on a SPECS PHOIBOS 150 electron spectrometer using the monochromated HeI radiation (21.2 eV). ICP-OES analysis of QD powders digested in nitric acid solution was performed with a PerkinElmer Optima 3200 RL. Device characterization The current voltage characteristics of solar cells under 100 mW cm −2 AM1.5 light provided by an Oriel Sol3A solar simulator were recorded using a Keithley 2400 sourcemeter, using appropriate aperture masks. The spectral external quantum efficiency of the cells was measured by recording the short-circuit current of the cells upon illumination with monochromatic light from a Newport Oriel apex illuminator–monochromator system. The monochromatic light intensity was measured using a Newport 818-IR and a 818-UV calibrated photodiode. Capacitance–voltage characteristics were recorded using an Agilent E4980A precision LCR meter. How to cite this article: Stavrinadis, A. et al . Heterovalent cation substitutional doping for quantum dot homojunction solar cells. Nat. Commun. 4:2981 doi: 10.1038/ncomms3981 (2013).